A variational eigenvalue solver on a photonic quantum processor Quantum computers promise to efficiently solve important problems that are intractable on a conventional computer. For quantum systems, where the physical dimension grows exponentially, finding the eigenvalues of certain operators is one such intractable problem and remains a fundamental challenge. The quantum phase estimation algorithm efficiently finds the eigenvalue of a given eigenvector but requires fully coherent evolution. Here we present an alternative approach that greatly reduces the requirements for coherent evolution and combine this method with a new approach to state preparation based on ansätze and classical optimization. We implement the algorithm by combining a highly reconfigurable photonic quantum processor with a conventional computer. We experimentally demonstrate the feasibility of this approach with an example from quantum chemistry—calculating the ground-state molecular energy for He–H + . The proposed approach drastically reduces the coherence time requirements, enhancing the potential of quantum resources available today and in the near future. In chemistry, the properties of atoms and molecules can be determined by solving the Schrödinger equation. However, because the dimension of the problem grows exponentially with the size of the physical system under consideration, exact treatment of these problems remains classically infeasible for compounds with more than 2–3 atoms [1] . Many approximate methods [2] have been developed to treat these systems, but efficient, exact methods for large chemical problems remain out of reach for classical computers. Beyond chemistry, the solution of large eigenvalue problems [3] would have applications ranging from determining the results of internet search engines [4] to designing new materials and drugs [5] . Recent developments in the field of quantum computation offer a way forward for determining efficient solutions of many instances of large eigenvalue problems that are classically intractable [6] , [7] , [8] , [9] , [10] , [11] , [12] . Quantum approaches to finding eigenvalues have previously relied on the quantum phase estimation (QPE) algorithm. The QPE algorithm offers an exponential speedup over classical methods and requires a number of quantum operations O ( p −1 ) to obtain an estimate with precision p (refs 13 , 14 , 15 , 16 , 17 , 18 ). In the standard formulation of QPE, one assumes the eigenvector | ψ › of a Hermitian operator is given as input and the problem is to determine the corresponding eigenvalue λ . The time the quantum computer must remain coherent is determined by the necessity of O ( p −1 ) successive applications of , each of which can require on the order of millions or billions of quantum gates for practical applications [17] , [19] , as compared to the tens to hundreds of gates achievable in the short term. Here we introduce an alternative to QPE that significantly reduces the requirements for coherent evolution. We have developed a reconfigurable quantum processing unit (QPU), which efficiently calculates the expectation value of a Hamiltonian ( ), providing an exponential speedup over exact diagonalization, the only known exact solution to the problem on a traditional computer. The QPU has been experimentally implemented using integrated photonics technology with a spontaneous parametric downconversion single-photon source and combined with an optimization algorithm run on a classical processing unit (CPU), which variationally computes the eigenvalues and eigenvectors of . By using a variational algorithm, this approach reduces the requirement for coherent evolution of the quantum state, making more efficient use of quantum resources, and may offer an alternative route to practical quantum-enhanced computation. Quantum expectation estimation The quantum expectation estimation (QEE) algorithm computes the expectation value of a given Hamiltonian for an input state | ψ ›. Any Hamiltonian may be written as for real h , where Roman indices identify the subsystem on which the operator acts, and Greek indices identify the Pauli operator, for example, α = x . Note that no assumption about the dimension or structure of the hermitian Hamiltonian is needed for this expansion to be valid. By exploiting the linearity of quantum observables, it follows that We consider Hamiltonians that can be written as a polynomial number of terms, with respect to the system size. This class of Hamiltonians encompasses a wide range of physical systems, including the electronic structure Hamiltonian of quantum chemistry, the quantum Ising Model, the Heisenberg Model [20] , [21] , matrices that are well approximated as a sum of n -fold tensor products [22] , [23] , and more generally any k -sparse Hamiltonian without evident tensor product structure (see Supplementary Methods for details). Thus, the evaluation of ‹ › reduces to the sum of a polynomial number of expectation values of simple Pauli operators for a quantum state | ψ ›, multiplied by some real constants. A quantum device can efficiently evaluate the expectation value of a tensor product of an arbitrary number of simple Pauli operators [23] . Therefore, with an n -qubit state we can efficiently evaluate the expectation value of this 2 n × 2 n Hamiltonian. One might attempt this using a classical computer by separately optimizing all reduced states corresponding to the desired terms in the Hamiltonian, but this would suffer from the N -representability problem, which is known to be intractable for both classical and quantum computers (it is in the quantum complexity class QMA-Hard [24] ). The power of our approach derives from the fact that quantum hardware can store a global quantum state with exponentially fewer resources than required by classical hardware, and as a result the N -representability problem does not arise. The expectation value of a tensor product of an arbitrary number of Pauli operators can be estimated by local measurement of each qubit [6] . Such independent measurements can be performed in parallel, incurring a constant cost in time. Furthermore, since these operators are normalized and finite-dimensional, their spectra are bounded. As a result, each can be estimated to a precision p of an individual element with coefficient h , which is an arbitrary element from the set of constants , at a cost of O (| h max | 2 Mp −2 ) repetitions. Here M is the number of terms in the decomposition of the Hamiltonian and h max is the coefficient with maximum norm in the decomposition of the Hamiltonian. The advantage of this approach is that the coherence time to make a single measurement after preparing the state is O (1). Conversely, the disadvantage of this approach with respect to QPE is the scaling in the total number of operations, as a function of the desired precision is quadratically worse ( O ( p −2 ) versus O ( p −1 )). Moreover, this scaling will also reflect the number of state preparation repetitions required, whereas in QPE the number of state preparation steps is constant. In essence, we dramatically reduce the coherence time requirement while maintaining an exponential advantage over the classical case, by adding a polynomial number of repetitions with respect to QPE. Quantum variational eigensolver The procedure outlined above replaces the long coherent evolution required by QPE by many short coherent evolutions. In both QPE and QEE we require a good approximation to the ground-state wavefunction to compute the ground-state eigenvalue, and we now consider this problem. Previous approaches have proposed to prepare ground states by adiabatic evolution [15] , or by the quantum Metropolis algorithm [25] , [26] . Unfortunately both of these require long coherent evolution. The quantum variational eigensolver (QVE) algorithm is a variational method to prepare the eigenstate and, by exploiting QEE, requires short coherent evolution. QEE and QVE and their relationship are shown in Fig. 1 and detailed in the Supplementary Methods . 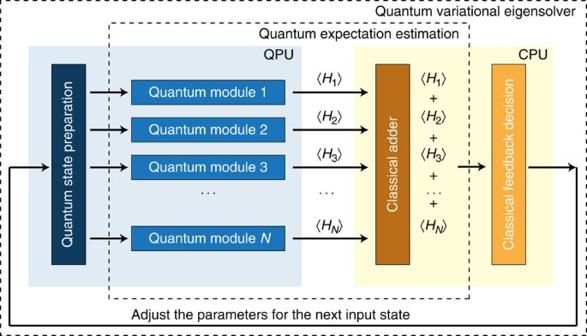Figure 1: Architecture of the quantum-variational eigensolver. In QEE, quantum states that have been previously prepared are fed into the quantum modules, which compute ‹i›, whereiis any given term in the sum defining. The results are passed to the CPU, which computes ‹›. In the quantum variational eigensolver, the classical minimization algorithm, run on the CPU, takes ‹› and determines the new state parameters, which are then fed back to the QPU. Figure 1: Architecture of the quantum-variational eigensolver. In QEE, quantum states that have been previously prepared are fed into the quantum modules, which compute ‹ i ›, where i is any given term in the sum defining . The results are passed to the CPU, which computes ‹ ›. In the quantum variational eigensolver, the classical minimization algorithm, run on the CPU, takes ‹ › and determines the new state parameters, which are then fed back to the QPU. Full size image It is well known that the eigenvalue problem for an observable represented by an operator can be restated as a variational problem on the Rayleigh–Ritz quotient [27] , [28] , such that the eigenvector | ψ › corresponding to the lowest eigenvalue is the | ψ › that minimizes By varying the experimental parameters in the preparation of | ψ › and computing the Rayleigh–Ritz quotient using QEE as a subroutine in a classical minimization, one may prepare unknown eigenvectors. At the termination of the algorithm, a simple prescription for the reconstruction of the eigenvector is stored in the final set of experimental parameters that define | ψ ›. If a quantum state is characterized by an exponentially large number of parameters, it cannot be prepared with a polynomial number of operations. The set of efficiently preparable states are therefore characterized by polynomially many parameters, and we choose a particular set of ansatz states of this type. Under these conditions, a classical search algorithm on the experimental parameters that define | ψ › needs only explore a polynomial number of dimensions—a requirement for the search to be efficient. One example of a quantum state parameterized by a polynomial number of parameters for which there is no known efficient classical implementation is the unitary coupled cluster ansatz [29] where |Φ› ref is some reference state, usually the Hartree Fock ground state, and T is the cluster operator for an N electron system, defined by where and higher-order terms follow logically. It is clear that by construction the operator ( T − T † ) is anti-hermitian, and exponentiation maps it to a unitary operator . For any fixed excitation level k , the reduced cluster operator is written as In general no efficient implementation of this ansatz has yet been developed for a classical computer, even for low-order cluster operators, due to the non-truncation of the BCH series [29] . However, this state may be prepared efficiently on a quantum device. The reduced anti-hermitian cluster operator ( T ( k ) − T ( k )† ) is the sum of a polynomial number of terms—namely, it contains a number of terms O ( N k ( M − N ) k ), where M is the number of single-particle orbitals. By defining an effective Hermitian Hamiltonian = i ( T ( k ) − T ( k )† ) and performing the Jordan–Wigner transformation to reach a Hamiltonian that acts on the space of qubits, , we are left with a Hamiltonian that is a sum of polynomially many products of Pauli operators. The problem then reduces to the quantum simulation of this effective Hamiltonian, , which can be done in polynomial time using the procedure outlined by Ortiz et al. [23] We note that while this state preparation procedure utilizes tools from quantum simulation, the total effective time of evolution is fixed by the expansion coefficients . This is in contrast to the normal difficulties encountered in QPE, where simulations must be carried out for times that are exponential in the desired bits of precision. While there is currently no known efficient classical algorithm based on these ansatz states, non-unitary coupled cluster ansatz is sometimes referred to as the ‘gold standard of quantum chemistry’ as it is the standard of accuracy to which other methods in quantum chemistry are often compared. The unitary version of this ansatz is thought to yield superior results to even this ‘gold standard’ [29] . Prototype demonstration We have implemented the QPU using integrated quantum photonics technology [30] . Our device, shown schematically in Fig. 2 , is a reconfigurable waveguide chip that can prepare and measure arbitrary two-bit pure states using several single-qubit rotations and one two-qubit entangling gate. The state is path-encoded using photon pairs generated via a spontaneous parametric downconversion process. State preparation and measurement in the Pauli basis is achieved by setting 8 voltage-driven phase shifters and counting photon detection events with silicon single-photon detectors [31] . 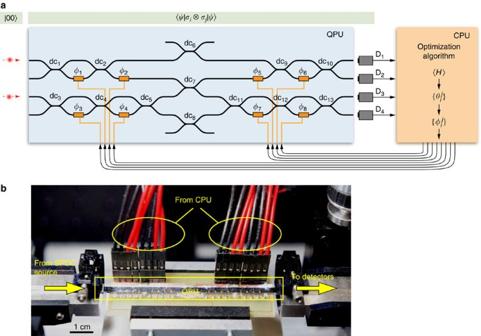Figure 2: Experimental implementation of our scheme. (a) Quantum-state preparation and measurement of the expectation values ‹ψ|σi⊗σj|ψ› are performed using a quantum photonic chip. Photon pairs, generated using spontaneous parametric downconversion, are injected into the waveguides encoding the |00› state. The state |ψ› is prepared using thermal phase shiftersφ1−8(orange rectangles) and one CNOT gate and measured using photon detectors. dc{1–4,9–13}(dc5–7) are 50% (30%) reflectivity directional couplers. Coincidence count rates from the detectors D1–4are passed to the CPU running the optimization algorithm. This computes the set of parameters for the next state and writes them to the quantum device. (b) A photograph of the QPU. Figure 2: Experimental implementation of our scheme. ( a ) Quantum-state preparation and measurement of the expectation values ‹ ψ | σ i ⊗ σ j | ψ › are performed using a quantum photonic chip. Photon pairs, generated using spontaneous parametric downconversion, are injected into the waveguides encoding the |00› state. The state | ψ › is prepared using thermal phase shifters φ 1−8 (orange rectangles) and one CNOT gate and measured using photon detectors. dc {1–4,9–13} (dc 5–7 ) are 50% (30%) reflectivity directional couplers. Coincidence count rates from the detectors D 1–4 are passed to the CPU running the optimization algorithm. This computes the set of parameters for the next state and writes them to the quantum device. ( b ) A photograph of the QPU. Full size image The ability to prepare an arbitrary two-qubit separable or entangled state enables us to investigate 4 × 4 Hamiltonians. For the experimental demonstration of our algorithm we choose a problem from quantum chemistry—namely, determining the bond dissociation curve of the molecule He–H + in a minimal basis. The full configuration interaction Hamiltonian for this system has dimension 4, and can be written compactly as The coefficients and were determined using the PSI3 computational package [32] and are tabulated in Supplementary Table 2 . In order to compute the bond dissociation of the molecule, we use QVE to compute its ground state for a range of values of the nuclear separation R . In Fig. 3 we report a representative optimization run for a particular nuclear separation, demonstrating the convergence of our algorithm to the ground state of ( R ) in the presence of experimental noise. 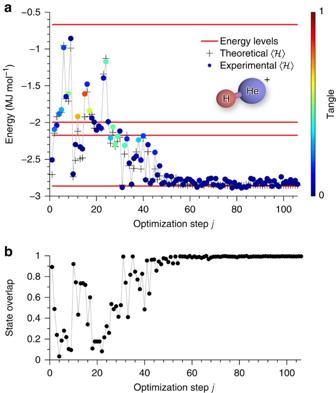Figure 3: Finding the ground state of He–H+for a specific molecular separationR=90 pm. (a) Experimentally computed energy ‹› (coloured dots) as a function of the optimization stepj. The colour represents the tangle (degree of entanglement) of the physical state, estimated directly from the state parameters. The red lines indicate the energy levels of(R). The optimization algorithm clearly converges to the ground state of the molecule, which has small but non-zero tangle. The crosses show the energy calculated at each experimental step, assuming an ideal quantum device. (b) Overlap |‹ψj|ψG› between the experimentally computed state |ψj› at each optimization stepjand the theoretical ground state of, |ψG›. Error bars are smaller than the data points. Further details are provided in the Methods section,Supplementary Table 1andSupplementary Methods. Figure 3a demonstrates the convergence of the average energy, while Fig. 3b demonstrates the convergence of the overlap |‹ ψ j | ψ G ›| of the current state | ψ j › with the target state | ψ G ›. The colour of each entry in Fig. 3a represents the tangle (absolute concurrence squared) of the state at that step of the algorithm. It is known that the volume of separable states is doubly exponentially small with respect to the rest of state space [33] . Thus, the ability to traverse non-separable state space increases the number of paths by which the algorithm can converge and will be a requirement for future large-scale implementations. Moreover, it is clear that the ability to produce entangled states is a necessity for the accurate description of general quantum systems where eigenstates may be non-separable—for example, the ground state of the He–H + Hamiltonian has small but not negligible tangle. Figure 3: Finding the ground state of He–H + for a specific molecular separation R =90 pm. ( a ) Experimentally computed energy ‹ › (coloured dots) as a function of the optimization step j . The colour represents the tangle (degree of entanglement) of the physical state, estimated directly from the state parameters . The red lines indicate the energy levels of ( R ). The optimization algorithm clearly converges to the ground state of the molecule, which has small but non-zero tangle. The crosses show the energy calculated at each experimental step, assuming an ideal quantum device. ( b ) Overlap |‹ ψ j | ψ G › between the experimentally computed state | ψ j › at each optimization step j and the theoretical ground state of , | ψ G ›. Error bars are smaller than the data points. Further details are provided in the Methods section, Supplementary Table 1 and Supplementary Methods . Full size image Repeating this procedure for several values of R , we obtain the bond dissociation curve, which is reported in Fig. 4 . After the computed energies have been corrected for experimental errors, the determination of the equilibrium bond length of the molecule was found to be R =92.3±0.1 pm, with a corresponding ground-state electronic energy of E =−2.865±0.008 MJ mol −1 . Full details of the correction for systematic errors and estimation of the uncertainty on E are reported in the Supplementary Methods . The corresponding theoretical curve shows the numerically exact energy derived from a full configuration interaction calculation of the molecular system in the same basis. More than 96% of the experimental data are within chemical accuracy with respect to the theoretical values. At the conclusion of the optimization, we retain full knowledge of the experimental parameters, which can be used for efficient reconstruction of the state | ψ › in the event that additional physical or chemical properties are required. 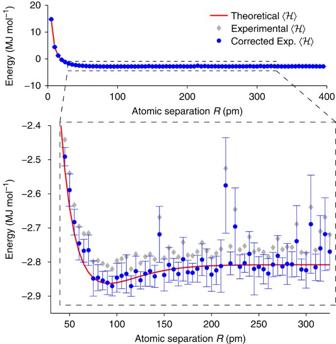Figure 4: Bond dissociation curve of the He–H+molecule. This curve is obtained by repeated computation of the ground-state energy (as shown inFig. 3) for several(R) values. The magnified plot shows that after correction for the measured systematic error the data overlap with the theoretical energy curve, and, importantly, we can resolve the molecular separation of minimal energy. Error bars show the standard deviation of the computed energy, as described in the Methods section. Figure 4: Bond dissociation curve of the He–H + molecule. This curve is obtained by repeated computation of the ground-state energy (as shown in Fig. 3 ) for several ( R ) values. The magnified plot shows that after correction for the measured systematic error the data overlap with the theoretical energy curve, and, importantly, we can resolve the molecular separation of minimal energy. Error bars show the standard deviation of the computed energy, as described in the Methods section. Full size image QEE uses relatively few quantum resources compared to QPE. Broadly speaking, QPE requires a large number of n -qubit quantum controlled operations to be performed in series—placing considerable demands on the number of components and coherence time—while the inherent parallelism of our scheme enables a small number of n -qubit gates to be exploited many times, drastically reducing these demands. Moreover, adding control to arbitrary unitary operations in practice is difficult, if not impossible, for current quantum architectures (although a proposed scheme to add control to arbitrary unitary operations has recently been demonstrated [34] ). To give a numerical example, the QPE circuit for a 4 × 4 Hamiltonian such as that demonstrated here would require at least 12 CNOT gates, while our method only requires one. We note that the resource saving provided by QEE incurs a cost of polynomial repetitions of the state preparation, as compared to the single copy required by QPE. In many cases (for example, our photonic implementation), repeated preparation of a state is not significantly harder than preparation of a single copy, requiring only a polynomial overhead in time without any modification of the device. In implementing QVE, the device prepares ansatz states that are defined by a polynomial set of parameters. This ansatz might be chosen based on knowledge of the physical system of interest (as for the unitary coupled cluster and typical quantum chemistry ansätze), thus determining the device design. However, our architecture allows for an alternative and potentially more promising approach, where the device is first constructed based on the available resources and we define the set of states that the device can prepare as the ‘device ansatz’. Due to the quantum nature of the device, this ansatz can be very distinct from those used in traditional quantum chemistry. With this alternative approach the physical implementation is then given by a known sequence of quantum operations with adjustable parameters—determined at the construction of the device—with a maximum depth fixed by the coherence time of the physical qubits. This approach, while approximate, provides a variationally optimal solution for the given quantum resources and may still be able to provide qualitatively correct solutions, just as approximate methods do in traditional quantum chemistry (for example, Hartree Fock). The unitary coupled cluster ansatz (equation (4)) provides a concrete example where our approach provides an exponential advantage over known classical techniques. For this ansatz, with as few as 40–50 qubits, one expects to manipulate a state that is not efficient to simulate classically, and can provide a solution superior to the classical gold standard, non-unitary coupled cluster. We have developed and experimentally implemented a new approach to solving the eigenvalue problem with quantum hardware. QEE shares with QPE the need to prepare a good approximation to the ground state, but replaces a single long coherent evolution by a number of shorter coherent calculations proportional to the number of terms in the Hamiltonian. While the effect of errors on each of these calculations is the same as in QPE, the reliance on a number of separate calculations makes the algorithm sensitive to variations in state preparation between the separate quantum calculations. This effect requires further investigation. The most general local Hamiltonian problem is QMA-complete [35] . However, under the reasonable assumption that a good approximation to the state can be prepared, our method and QPE can both efficiently estimate the energy of the state, and it is in this setting that we compare them. In QVE, we experimentally implemented a ground-state preparation procedure through a direct variational algorithm on the control parameters of the quantum hardware. The prepared state could be utilized in either QEE 1 or QPE if desired. Larger calculations will require a choice of ansatz, for which there are two possibilities. One could experimentally implement chemically motivated ansatz such as the unitary coupled cluster method. Alternatively, one could pursue those ansätze that are most easy to implement experimentally—creating a new set of device ansatz states that would require classification in terms of their overlap with chemical ground states. Such a classification would be a good way to determine the value of a given experimental advance—for ground-state problems it is best to focus limited experimental resources on those efforts that will most enhance the overlap of preparable states with chemical ground states. In addition to the above issues, which we leave to future work, an interesting avenue of research is to ask whether the conceptual approach described here could be used to address other intractable problems with quantum-enhanced computation. Examples that can be mapped to the ground-state problem, and where the N -representability problem does not occur, include search engine optimization and image recognition. It should be noted that the approach presented here requires no control or auxiliary qubits, relying only on measurement techniques that are already well established. For example, in the two-qubit case, these measurements are identical to those performed in Bell inequality experiments. Quantum simulators with only a few tens of qubits are expected to outperform the capabilities of conventional computers, not including open questions regarding fault tolerance and errors/precision. Our scheme would allow such devices to be implemented using dramatically less resources than the current best known approach. Classical optimization algorithm For the classical optimization step of our integrated processor we implemented the Nelder–Mead (NM) algorithm [36] , a simplex-based direct search (DS) method for unconstrained minimization of objective functions. Although in general NM can fail because of the deterioration of the simplex geometry or lack of sufficient decrease, the convergence of this method can be greatly improved by adopting a restarting strategy. Although other DS methods, such as the gradient descent, can perform better for smooth functions, these are not robust to the noise, which makes the objective function non-smooth under experimental conditions. NM has the ability to explore neighbouring valleys with better local optima, and likewise this exploring feature usually allows NM to overcome non-smoothnesses. We verified that the gradient descent minimization algorithm is not able to converge to the ground state of our Hamiltonian under the experimental conditions, mainly due to the Poissonian noise associated with our photon source and the accidental counts of the detection system, while NM converged to the global minimum in most optimization runs. Mapping from the state parameters to the chip phases The set of phases { θ i }, which uniquely identifies the state | ψ ›, is not equivalent to the phases that are written to the photonic circuit { φ i }, since the chip phases are also used to implement the desired measurement operators σ α ⊗ σ β . Therefore, knowing the desired state parameters and measurement operator we compute the appropriate values of the chip phases on the CPU at each iteration of the optimization algorithm. The algorithm for finding the state parameters { θ i } for an arbitrary two-qubit state is described in the Methods. These phases are then applied to the CNOT-MZ chip using φ 1,2,3,4,7,8 . Here φ 7,8 are modified to account for the choice of measurment setting at the target qubit. (Any single-qubit projective measurement can be performed using an MZI together with two phase shifters.) The measurement setting for the control qubit is implemented using φ 5,6 . Estimation of the error on ‹ › We performed measurements of the statistical and systematic errors that affect our computation of ‹ ›. Statistical errors Statistical errors due to the Poissonian noise associated with single-photon statistics are intrinsic to the estimation of expectation values in quantum mechanics. These errors can be arbitrarily reduced at a sublinear cost of measurement time (that is, efficiently) since the magnitude of error is proportional to the square root of the count rate. We experimentally measured the standard deviation of an expectation value ‹ i › for a particular state using 50 trials. The total average coincidence rate was ~1,500 s −1 . The standard deviation was found to be 37 kJ mol −1 , which is comparable to the error observed in the measurement of the ground-state energy shown in Fig. 4 . The minima of the potential energy curve was determined by a generalized least squares procedure to fit a quadratic curve to the experimental data points in the region R =(80, 100) pm, as is common in the use of trust region searches for minima [37] , using the inverse experimentally measured variances as weights. Covariances determined by the generalized least squares procedure were used as input to a Monte Carlo sampling procedure to determine the minimum energy and equilibrium bond distance as well as their uncertainties assuming Gaussian random error. The uncertainties reported represent standard deviations. Sampling error in the Monte Carlo procedure was 3 × 10 −4 pm for the equilibrium bond distance and 3 × 10 −8 MJ mol −1 for the energy. In Fig. 4 , the large deviations from the theoretical line result from the coincidental impact of noise resulting in premature optimization termination. These points could have been rerun or eliminated using the prior knowledge of smoothness of the dissociation curve. However, to accurately portray the performance of the algorithm exactly as described, with no expert interference, these points are retained. Systematic errors In all the measurements described above we observed a constant and reproducible small shift, ε=50 kJ mol −1 , of the expectation value with respect to the theoretical value of the energy. There are at least three effects that contribute to this systematic error. Firstly, the downconversion source that we use in our experiment does not produce the pure two-photon state that is required for high-fidelity quantum interference. In particular, higher-order photon number terms and, more significantly, photon distinguishability both degrade the performance of our entangling gate and thus the preparation of the state | ψ ›. This results in a shift of the measured energy ‹ ψ | | ψ ›. Higher-order terms could be effectively eliminated by use of true single-photon sources (such as quantum dots or nitrogen vacancy centers in diamond), and there is no fundamental limit to the degree of indistinguishability that can be achieved through improved state engineering. Secondly, imperfections in the implementation of the photonic circuit also reduce the fidelity with which | ψ › is prepared and measured. Small deviations from designed beamsplitter reflectivities and interferometer path lengths, as well as imperfections in the calibration of voltage-controlled phase shifters used to manipulate the state, all contribute to this effect. However, these are technological limitations that can be greatly improved in future realizations. Finally, unbalanced input and output coupling efficiency also results in skewed two-photon statistics, again shifting the measured expectation value of ‹ ›. Another systematic effect that can be noted in Fig. 4 is that the magnitude of the error on the experimental estimation of the ground-state energy increases with R . This is due to the fact that as R increases the first and second excited eigenstates of this Hamiltonian become degenerate, resulting in increased difficulty for the classical minimization, generating mixtures of states that increases the overall variance of the estimation. Quantum-state fidelity In a previous work [31] , we measured the average state fidelity of states generated by the CNOT gate, estimated by quantum process tomography, to be 0.873±0.001. The average quantum-state fidelity over four Bell states was 0.93. The average fidelity across 995 configurations (equivalent to many truth tables in many bases) was 0.990±0.009, with 96% of configurations producing photon statistics with f >0.97. Count rate In our experiment the mean count rate, which directly determines the statistical error, was ~2,000–4,000 twofold events per measurement. The expectation value of a given Hamiltonian was reconstructed at each point from four two-qubit Pauli measurements. For the bond dissociation curve we measured about 100 points per optimization run. In the full dissociation curve we found the ground states of 79 Hamiltonians. The full experiment was performed in about 158 h. State preparation is relatively fast, requiring a few milliseconds to set the phases on the chip. However, 17 s is required for cooling the chip, resulting in a duty cycle of ~5%. The purpose of this is to overcome theinstability of the fibre-to-chip coupling due to thermal expansion of the chip during operation. This will not be an issue in future implementations, where fibres will be permanently fixed to the chip’s facets. Moreover, the thermal phase shifters used here will also likely be replaced by alternative technologies based on the electro-optic effect. Brighter single-photon sources will considerably reduce the measurement time. How to cite this article: Peruzzo, A. et al. A variational eigenvalue solver on a photonic quantum processor. Nat. Commun. 5:4213 doi: 10.1038/ncomms5213 (2014).